ASPM regulates symmetric stem cell division by tuning Cyclin E ubiquitination We generate a mouse model for the human microcephaly syndrome by mutating the ASPM locus, and demonstrate a premature exhaustion of the neuronal progenitor pool due to dysfunctional self-renewal processes. Earlier studies have linked ASPM mutant progenitor excessive cell cycle exit to a mitotic orientation defect. Here, we demonstrate a mitotic orientation-independent effect of ASPM on cell cycle duration. We pinpoint the cell fate-determining factor to the length of time spent in early G1 before traversing the restriction point. Characterization of the molecular mechanism reveals an interaction between ASPM and the Cdk2/Cyclin E complex, regulating the Cyclin activity by modulating its ubiquitination, phosphorylation and localization into the nucleus, before the cell is fated to transverse the restriction point. Thus, we reveal a novel function of ASPM in mediating the tightly coordinated Ubiquitin- Cyclin E- Retinoblastoma- E2F bistable-signalling pathway controlling restriction point progression and stem cell maintenance. Maintenance of stem cell populations employs intricate diverse mechanisms committed to balance cell division and differentiation by utilizing intrinsic and extrinsic regulatory factors. Understanding the mechanisms that promote stem cell maintenance should offer new opportunities to counter degenerative diseases and to use these cells for therapeutic purposes. An informative strategy is to detect genes that play central roles in pathways that regulate the maintenance and self-renewal of stem cells. The current study describes a newly generated mouse model for the human microcephaly syndrome [1] , [2] targeted at the ASPM gene. It establishes that an overall reduced brain size of ASPM mutant mice with distinct radial thinning of the cortical wall was due to premature exhaustion of the neural progenitor cell (NPC) reservoir owing to dysfunctional self-renewing divisions. Molecular mechanisms have evolved to regulate embryonic NPC expansion ensuring the maintenance of sufficient progenitors to meet the exponential demand for subsequent born neurons [3] , [4] . It has been suggested that the ASPM gene has undergone positive selection during hominid development that instigated the dramatic evolutionary increase in cortical neurons [1] , [5] , [6] . The ASPM localization to the minus ends of central spindle microtubules, centrosomes and spindle poles has been central to its functional analyses [7] , [8] . In response to external pulling forces, ASPM, complexed with LIN-5 and calmodulin at the poles, directs spindle alignment according to cues from the cell subcortex [9] . Mice in which ASPM is downregulated showed abnormal cleavage plane orientation of mitotic NPC [10] and a concurrent decline in symmetric progenitor divisions. However, it is controversial whether cleavage plane angle is the primary determinant mediating mammalian progenitor/stem cell divisions [3] . Mice mutant for the polarity determinant aPKCλ exhibited impeded mitotic cell divisions due to disrupted apical adherens junctions. Yet, corticogenesis and brain size were normal [11] . Depletion of LGN , a non-centrosomal determinant of spindle orientation, caused randomized cell division and apical progenitor displacement. Nevertheless, progenitor pool and cortex development were intact [12] . Recent data have shown that mouse and primate mitotic spindle size asymmetry is a key component of asymmetric cell division in the cerebral cortex [13] independently of spindle orientation [14] . Despite that, abnormal cleavage orientation remains the exclusive explanation for the declines in symmetric progenitor divisions in ASPM downregulated mice [10] . The widely accepted G1- phase length hypothesis [3] , [15] , [16] , [17] uses the progressive lengthening of the G1-phase from 3 to 12 h in the mouse cortex [18] to address the apparent inconsistency between an increasing frequency of NPC undergoing neurogenic-differentiative divisions despite steady state proportions of tilted dividing NPC during corticogenesis. The premise of the hypothesis is that regardless of division orientation, if the G1-phase is sufficiently long for the cell to receive and process intrinsic or extrinsic differentiative signals, then the daughter cells will exit the cell cycle (CC). Its support comes from studies that triggered premature neurogenic divisions by artificially lengthening NPC-CC [19] , [20] , [21] . Conversely, forced shortening of the NPC-CC promoted symmetric proliferative cell divisions [21] , [22] , [23] , [24] . G1 is considered to be a critical period during which cells decide whether to progress to S-phase, enter quiescence or differentiate. In fact, it has been proposed that G1 shortening shields pluripotent ES cells from differentiation inducing cues. ES cell insensitivity to differentiating signals due to a brief G1 is a result of excessive levels of constitutively active Cyclin E/Cdk2 complex resulting in hyperphosphorylation of retinoblastoma (RB) [25] , [26] . As development proceeds, multipotent stem cells go through a lengthening of G1, which permits increased checkpoints and cell extrinsic regulation. In addition to mitotic orientation dependence, a novel mechanism by which ASPM regulates NPC division is presented here. By interaction with Cyclin E/Cdk2, ASPM controls Cyclin E abundance through regulating its ubiquitin-dependent proteolysis. Shown here is that the ASPM− Ubiquitin− Cyclin E− RB− E2F pathway regulates numerous aspects of NPC-CC progression, including mitosis duration and passage through the G1 restriction point. Exogenous Cyclin E or proteasome inhibitor administered to the developing ASPM null cortex rescue its NPC aberrant CC timing and fate determination, but not the abnormal mitotic cleavage orientation, providing conclusive evidence linking the mode of progenitor division to the time residing within the early part of G1. Microcephalic characteristics of ASPM mutant mice To investigate the role of ASPM in brain development, an ASPM truncating mutation was fashioned by insertion of an ires-cre-neo cassette ( Supplementary Fig. 1a ). Northern and western blotting analyses ( Supplementary Fig. 1b ) confirmed the predicted truncation of ASPM mRNA and protein in homozygous mutant mice (henceforth referred to as ASPM Δ ). ASPM Δ mice are viable, born in Mendelian ratios and show a fully penetrant 20% smaller wet brain weight as embryo, continuing throughout life with a particular reduction in cortical dimension ( Fig. 1a–c and Supplementary Fig. 1c–g ) [8] . ASPM Δ adults are similar in body weight to WT and heterozygous littermates ( Fig. 1d ) therefore they maintain abnormally low brain-to-body weight ratios, which is a hallmark of the microcephalic phenotype in humans. 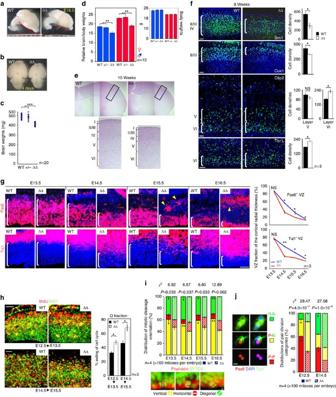Figure 1: Thinning of outer cortical layers owing to premature exhaustion of NPC pool because of improper division. (a,b) Dorsal and side views of embryo and newborn brains. (c) Distribution of 10 weeks brain weights ofASPMΔmice and their WT and heterozygous littermates (n=10 each gender). (d) Mean brain to body ratios and body weights. (e,f) Matching adult coronal cortical sections stained for H&E, Layer VI Tbr1−, layers V–VI Ctip2−, layers II-IV Brn1−, and layers II–III Cux1− neurons. Right bar graphs (f) demonstrate the cell density within each population. (g) Coronal cortical sections stained for Pax6 neural progenitor marker or Tuj1, which expressed exclusively in differentiated neurons. Right, graphs demonstrating the relative size of the Pax6+− or Tuj1−-regions, expressed as fractions of the whole cortical wall radial thickness. For further discussion on the displaced Pax6+foci located outside the VZ in E15.5 and E16.5ASPMΔcortices (arrowheads), seeSupplementary Note 1. (h) Coronal cortical sections 24 h after BrdU pulse stained for BrdU and Ki67. The fractions of cells that exited the CC and were no longer dividing (BrdU+/Ki67−; red) presented as the percentage of total BrdU+cells (red+yellow). (i) Representative axes of anaphase/telophase cortical mitotic divisions (white lines). The cleavage plane was defined as the orthogonal plane bisecting the line between the centers of each chromosome stained with SYTOX. Cell membrane was stained for phalloidin. (j) Panels show pairs of cells generated from a single progenitor 24 h after plating, stained for Pax6 and Tuj1. P-P; symmetric proliferative division produces a pair of precursors. P-N; asymmetric neurogenic division generates one precursor and one neuron. N-N; symmetric terminal neurogenic division generates two neurons. All graphs display mean±s.e.m.Χ2-squared statistical analyses show that distribution ofASPMΔmitotic orientation and distribution ofASPMΔmode of division are significantly different than control. *P<0.05, **P<0.005, ***P<0.001 by Student’st-test. Scale bars, 5 μm (i), 20 μm (j), 50 μm (f–h). Figure 1: Thinning of outer cortical layers owing to premature exhaustion of NPC pool because of improper division. ( a , b ) Dorsal and side views of embryo and newborn brains. ( c ) Distribution of 10 weeks brain weights of ASPM Δ mice and their WT and heterozygous littermates ( n =10 each gender). ( d ) Mean brain to body ratios and body weights. ( e , f ) Matching adult coronal cortical sections stained for H&E, Layer VI Tbr1−, layers V–VI Ctip2−, layers II-IV Brn1−, and layers II–III Cux1− neurons. Right bar graphs ( f ) demonstrate the cell density within each population. ( g ) Coronal cortical sections stained for Pax6 neural progenitor marker or Tuj1, which expressed exclusively in differentiated neurons. Right, graphs demonstrating the relative size of the Pax6 + − or Tuj1 − -regions, expressed as fractions of the whole cortical wall radial thickness. For further discussion on the displaced Pax6 + foci located outside the VZ in E15.5 and E16.5 ASPM Δ cortices (arrowheads), see Supplementary Note 1 . ( h ) Coronal cortical sections 24 h after BrdU pulse stained for BrdU and Ki67. The fractions of cells that exited the CC and were no longer dividing (BrdU + /Ki67 − ; red) presented as the percentage of total BrdU + cells (red+yellow). ( i ) Representative axes of anaphase/telophase cortical mitotic divisions (white lines). The cleavage plane was defined as the orthogonal plane bisecting the line between the centers of each chromosome stained with SYTOX. Cell membrane was stained for phalloidin. ( j ) Panels show pairs of cells generated from a single progenitor 24 h after plating, stained for Pax6 and Tuj1. P-P; symmetric proliferative division produces a pair of precursors. P-N; asymmetric neurogenic division generates one precursor and one neuron. N-N; symmetric terminal neurogenic division generates two neurons. All graphs display mean±s.e.m. Χ 2 -squared statistical analyses show that distribution of ASPM Δ mitotic orientation and distribution of ASPM Δ mode of division are significantly different than control. * P <0.05, ** P <0.005, *** P <0.001 by Student’s t -test. Scale bars, 5 μm ( i ), 20 μm ( j ), 50 μm ( f – h ). Full size image Premature exhaustion of cortical ASPM Δ NPC pool Histological analysis of adult ASPM Δ brains showed distinct thinning of the cortex that stems from a pronounced reduction of the superficial, later born layers II–IV ( Fig. 1e,f ). The substantial decrease in superficial layers corresponded to an increase in older and deeper layer VI cells ( Fig. 1f ). Although ASPM is predominantly expressed in the proliferating ventricular and subventricular zones (VZ and SVZ) along the four ventricles of the embryonic CNS [1] , [8] ( Supplementary Fig. 1h ), the cortical irregularities evolved in the absence of apparent alterations of VZ/SVZ growth fraction (GF), cell death and neural migration ( Supplementary Figs 1i–k and 2a ). The expanded deep layer and reduced superficial layers point to premature increase in cell output at the expense of the proliferative pool and subsequent later born neuron production. Accordingly, Fig. 1g evidences a sharper progressive reduction of the ASPM Δ NPC compartment at mid-to-late corticogenesis ( Supplementary Fig. 2b ), and Fig. 1h substantiates premature withdrawal of cells due to increased probability of VZ-NPC cell-cycle exit ( Q uiescence fraction) at the expense of the proportion of daughter cells that re-enter the cell cycle ( P roliferative fraction) [18] . Thus, ASPM is required to facilitate NPC advance into S-phase rather than exiting from active CC, and its deficiency results in abnormally increased kinetics of the P to Q shift. Irregular neurogenic to proliferative division ratio In accordance with previous observations reported from knock down experiments [10] , ASPM truncation caused a shift towards horizontal and oblique mitotic cleavage planes with a consequent considerable decrease in the proportion of basal mitoses with apicobasal cleavage planes ( Fig. 1i ). Although horizontal cleavage planes typically generate asymmetric cell fates, with one P daughter cell and a Q neuron [27] , [28] , [29] , irregular cleavage orientation of ASPM Δ basal mitoses is neither sufficient to explain the generation of excessive neural progeny ( Fig. 1h ), nor the accelerated depletion of the progenitor pool ( Fig. 1g ). As illustrated in Fig. 1i , throughout both WT and ASPM Δ corticogenesis, proportions are maintained overtime but differ between genotypes. Therefore, the progressively increasing Q fraction reported here ( Fig. 1h ) and by others [18] , [29] requires an additional mechanism unrelated to cleavage plane orientation for mediating asymmetric and symmetric divisions. For this reason, ASPM’s role in cell fate decisions was examined in clonal pair-cell assay. Scoring the fate of a single precursor’s first division following isolation from the embryonic cortex revealed that ASPM Δ NPC carried out significantly more P-N asymmetric-neurogenic divisions in young E12.5 embryos, and more N-N symmetric-neurogenic divisions in older E14.5 embryos, always at the expense of P-P symmetric-proliferative divisions ( Fig. 1j and Supplementary Fig. 2c ). Hence, ASPM is necessary to maintain symmetric P-P proliferative divisions of NPC even in the absence of a specific structural niche. Impaired cell cycle of ASPM Δ NPC During typical corticogenesis, the progressive increase in neuron production (Q) ( Fig. 1h ) and frequency of neurogenic divisions (P-N and N-N) ( Fig. 1j ) coincides with a progressive lengthening of the CC, mainly due to a slow down of the G1-phase [18] . In fact, converging observations suggested a link between CC kinetics and the mode of NPC division [15] , [16] , [19] , [20] , [21] , [22] , [30] , [31] ( Supplementary Fig. 3 ). Correspondingly, three distinct analyses pointed to impaired CC progression of ASPM Δ cortical NPC. First, similar to previously reported ASPM siRNA knockdown experiments [32] , [33] , in response to growth factors the average clonal size of E14.5 telencephalic derived ASPM Δ neurospheres was significantly smaller ( Fig. 2a ), indicting an impaired capacity to respond to proliferative signals. Also, secondary and tertiary neurosphere formation (from single dissociated primary and secondary spheres) showed significant impairment in ASPM Δ NPC self-renewal capacity ( Fig. 2b ). To reinforce the in vitro observation, an in vivo display of impaired CC was provided by analysis of the neurogenetic interval duration. 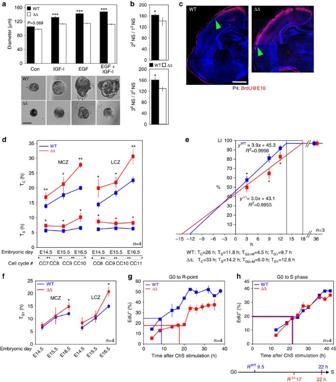Figure 2: ASPM is critical for proper CC kinetics. (a) Phase contrast microscopy of secondary neurospheres. (n=5 embryos, ≥100 spheres per embryo). (b) Self-renewal capacity of primary and secondary neurospheres (NS) cultured for 5 days without growth factors. (n=4 independent experiments, 80 subcloned spheres per experiment). (c) Coronal cortical sections demonstrating the lateral extent of the spread (termination wave front) at the border between the area of the VZ that continues to produce neurons (BrdU+) and the area in which the VZ have involuted and no longer proliferates (BrdU−), mapped in the grey matter with respect to cortical cytoarchitectonic fields. (d) VZ-NPC TCand TS. MCZ and LCZ, medial and lateral cortical zones, respectively. (e) Best-fit plots of LI versus survival time for E16.5ASPMΔand WT embryos rose precipitously during BrdU administration at 2 h intervals, irrespective of genotype until reaching saturation at the GF value. LI values were significantly greater in WT embryos, indicating faster BrdU labelling. A 2 × 3 factor ANOVA (groups × survival times) established a significant main effect of groups on LI (F=114.01;P<0.0001). Accordingly, the TCduration ofASPMΔSVZ progenitors was 7 h longer and TSwas 2.4 h longer. TG2+Mwas deduced fromSupplementary Fig. 8c, and TG1=TC—TS—TG2+M. (f) Plots of VZ-NPC TG1. (g) R-point analysis. Freshly isolated serum starved synchronized E12.5 telencephalic NPC were stimulated with chicken serum (ChS) for the indicated times. The serum was removed, and cells were incubated with serum free medium and EdU. Percentage of EdU+cells plotted versus stimulus duration. (h) S-phase entry analysis. Serum starved synchronized E12.5 NPC were continuously stimulated with ChS and EdU for the indicated times. Results were plotted as inf. Chronological representation of the G0 to R-point to S-phase intervals is shown. All graphs display mean±s.e.m. *P<0.05, **P<0.005, ***P<0.001 by Student’st-test. Scale bars, 100 μm (a), 500 μm (c). Figure 2c shows singly BrdU labelled (at E16) matching P4 coronal cortical planes in which the cortical termination wave front of ASPM Δ mutant appeared laterally displaced (arrows). Since the initiation and termination ‘wave fronts’ of neural production advances along the rostrolateral to caudomedial axis of the cortical hemisphere [34] , monitoring the transverse neurogenetic termination gradient allows comparison of neurogenetic interval durations between developing cortices. Accordingly, the laterally displaced ASPM Δ termination wave front indicates an extended corticogenesis. Lastly, ASPM Δ NPC exhibited delayed succession of an internal clockwise developmental sequence, shown by tracking the expression and cellular localization of the Cux1 and Brn1 transcription factors ( Supplementary Fig. 4 ). Figure 2: ASPM is critical for proper CC kinetics. ( a ) Phase contrast microscopy of secondary neurospheres. ( n =5 embryos, ≥100 spheres per embryo). ( b ) Self-renewal capacity of primary and secondary neurospheres (NS) cultured for 5 days without growth factors. ( n =4 independent experiments, 80 subcloned spheres per experiment). ( c ) Coronal cortical sections demonstrating the lateral extent of the spread (termination wave front) at the border between the area of the VZ that continues to produce neurons (BrdU + ) and the area in which the VZ have involuted and no longer proliferates (BrdU − ), mapped in the grey matter with respect to cortical cytoarchitectonic fields. ( d ) VZ-NPC T C and T S . MCZ and LCZ, medial and lateral cortical zones, respectively. ( e ) Best-fit plots of LI versus survival time for E16.5 ASPM Δ and WT embryos rose precipitously during BrdU administration at 2 h intervals, irrespective of genotype until reaching saturation at the GF value. LI values were significantly greater in WT embryos, indicating faster BrdU labelling. A 2 × 3 factor ANOVA (groups × survival times) established a significant main effect of groups on LI ( F =114.01; P <0.0001). Accordingly, the T C duration of ASPM Δ SVZ progenitors was 7 h longer and T S was 2.4 h longer. T G2+M was deduced from Supplementary Fig. 8c , and T G1 =T C —T S —T G2+M . ( f ) Plots of VZ-NPC T G1 . ( g ) R-point analysis. Freshly isolated serum starved synchronized E12.5 telencephalic NPC were stimulated with chicken serum (ChS) for the indicated times. The serum was removed, and cells were incubated with serum free medium and EdU. Percentage of EdU + cells plotted versus stimulus duration. ( h ) S-phase entry analysis. Serum starved synchronized E12.5 NPC were continuously stimulated with ChS and EdU for the indicated times. Results were plotted as in f . Chronological representation of the G0 to R-point to S-phase intervals is shown. All graphs display mean±s.e.m. * P <0.05, ** P <0.005, *** P <0.001 by Student’s t -test. Scale bars, 100 μm ( a ), 500 μm ( c ). Full size image To precisely measure in vivo CC duration, two assays were employed; double IdU/BrdU labelling procedure ( Supplementary Fig. 5 ) and cumulative labelling index (LI) approach ( Supplementary Fig. 6 ). The measurements revealed that overall CC length (T C ) was significantly longer in both ASPM Δ VZ-NPC ( Fig. 2d and Supplementary Tables 1 and 2 ) and in ASPM Δ SVZ progenitors ( Fig. 2e ). Surprisingly, neither FACS analyses nor Ki67 staining highlighted any particular phase contributing disproportionately to the considerably lengthened T C ( Supplementary Fig. 7 ), suggesting that all CC phases are comparatively extended in ASPM Δ germinal layers. Accordingly, the double IdU/BrdU labelling and cumulative LI techniques proved that duration of S-phase (T S ) in both germinal layers were significantly longer in ASPM Δ NPC ( Fig. 2d,e ). Next, the combined length of G2− and M-phases (T G2+M ) was determined by monitoring the percentage of labelled mitoses demonstrating that T G2+M of mutant NPC was invariantly 1.5 h longer in both germinal layers ( Supplementary Fig. 8 and Supplementary Tables 3 and 4 ). On the other hand, initial ASPM Δ G1-phase duration was not significantly longer. Only at E16.5 did the trend become significant in both VZ− and SVZ-NPC ( Fig. 2e,f and Supplementary Table 2 ). This result departs unexpectedly from the widely accepted relationship between G1 duration and the mode of NPC division [15] , as ASPM Δ NPC displayed increased neurogenic divisions earlier then E16.5 ( Fig. 1h,j ). Therefore, kinetics of G1 during early corticogenesis were further explored, particularly the passage through restriction (R)-point from mitogen-dependent early to mitogen-independent late G1-phases [35] . Timing the passage through the R-point along the G0 to S-phase interval of cultured synchronized NPC ( Supplementary Fig. 9a ) revealed that the early G1 of ASPM Δ NPC was 7.5 h longer ( Fig. 2g ). Notably, the defect in R-point regulation did not account to an overall increase in G1 duration, since kinetics of S phase entries ( Supplementary Fig. 9b ) were nearly identical between ASPM Δ and WT ( Fig. 2h ). Thus, the passage from the intrinsic and extrinsic signal-dependent early G1 to mitogen-independent late G1 is inefficient in ASPM Δ NPC. Delayed Cyclin E accumulation and sequential phosphorylation To understand the molecular mechanism underlying the ASPM regulation of R-point transition, protein levels of the transition main regulators were compared between ASPM Δ and WT NPC. ASPM Δ NPC displayed normal levels of Cdk2 and relatively similar levels and expression pattern of the early G1 regulator Cyclin D1 ( Fig. 3a and Supplementary Fig. 10a ). On the other hand, levels of the late G1 regulator, Cyclin E, were significantly downregulated in ASPM Δ NPC ( Fig. 3b ) corresponding with decreased activity of the Cyclin E/Cdk2 complex ( Fig. 3c ). Equal Cyclin D1 kinase activity between ASPM Δ and WT NPC reflected the comparable Cyclin D1 protein levels ( Fig. 3a,c ). Moreover, unchanged Cyclin D1 kinase activity proved that the increased p27 levels ( Fig. 3a ) did not inhibit Cyclin D1/Cdk(4/6) activity in ASPM Δ NPC. For comprehensive discussion into ASPM indirect regulation of p27 levels see Supplementary Fig. 10 . 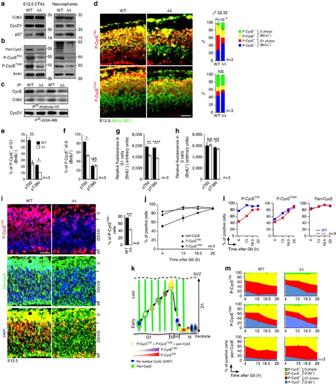Figure 3: ASPM regulates P-Cyclin E abundance and distribution. (a,b) Lysates of E12.5 telencephalons and primary neurospheres analysed for endogenous protein levels. The neurosphere low molecular weight Cyclin E is due to protease or alternative splicing processing69. (c) Assessment of Cyclin/Cdk complex activities. (d) E12.5 embryos were BrdU-pulse labelled for 30 min. Coronal cortical sections were stained for BrdU and the indicated phosphorylated Cyclin E. Cell counts excluded mitotic cells. Because cells between M− and S-phase zones are overwhelming in the G1, all BrdU-negative cells were considered in G1, and were classified as P-Cyclin E+(red) or P-Cyclin E−(blue; DAPI). S-phase BrdU-positive cells were sorted as P-Cyclin E+(yellow) and P-Cyclin E−(green). (e,f) Charts demonstrating the proportions of indicated P-Cyclin E+NPC within G1− (BrdU−) and S− (BrdU+) cell fractions, respectively. (g,h) Charts demonstrating quantification of mean relative fluorescence intensity per cell of P-Cyclin ET62and P-Cyclin ET380staining in G1− and S-phase cells. (i) E12.5 coronal cortical sections stained for total pan-Cyclin E and P-Cyclin ET62. Graph demonstrates the P-Cyclin ET62+cell density within the VZ. Cell counts excluded mitotic cells. Blue (DAPI) and red co-staining demonstrates nuclear P-Cyclin ET62+localization. (j) Freshly isolated serum starved synchronized E12.5 NPC were stimulated with ChS for the indicated times and stained for the indicated P-Cyclin E. Percentage of P-Cyclin E+WT NPC plotted versus stimulus duration. (k) Interpretation of 3d-3j summarized as a cartoon representing cellular localization of Cyclin E along the inter-nuclear movement of WT VZ-NPC. For further discussion seeSupplementary Note 2. (l) Comparison between WT− andASPMΔ-NPC shown in 3j. (m) The NPC described in 3l were also EdU pulse labeled at the indicated times. Percentage of EdU+/P-Cyclin E+cells plotted versus stimulus duration. For high resolution of panelsdandi, seeSupplementary Fig. 11. Graphs represent quantified three mice and four sections per mouse. All graphs display mean±s.e.m. *P<0.05, **P<0.01, ***P<0.0005, ****P<0.00005 by Student’st-test. Scale bars, 50 μm. Figure 3: ASPM regulates P-Cyclin E abundance and distribution. ( a , b ) Lysates of E12.5 telencephalons and primary neurospheres analysed for endogenous protein levels. The neurosphere low molecular weight Cyclin E is due to protease or alternative splicing processing [69] . ( c ) Assessment of Cyclin/Cdk complex activities. ( d ) E12.5 embryos were BrdU-pulse labelled for 30 min. Coronal cortical sections were stained for BrdU and the indicated phosphorylated Cyclin E. Cell counts excluded mitotic cells. Because cells between M− and S-phase zones are overwhelming in the G1, all BrdU-negative cells were considered in G1, and were classified as P-Cyclin E + (red) or P-Cyclin E − (blue; DAPI). S-phase BrdU-positive cells were sorted as P-Cyclin E + (yellow) and P-Cyclin E − (green). ( e , f ) Charts demonstrating the proportions of indicated P-Cyclin E + NPC within G1− (BrdU − ) and S− (BrdU + ) cell fractions, respectively. ( g , h ) Charts demonstrating quantification of mean relative fluorescence intensity per cell of P-Cyclin E T62 and P-Cyclin E T380 staining in G1− and S-phase cells. ( i ) E12.5 coronal cortical sections stained for total pan-Cyclin E and P-Cyclin E T62 . Graph demonstrates the P-Cyclin E T62+ cell density within the VZ. Cell counts excluded mitotic cells. Blue (DAPI) and red co-staining demonstrates nuclear P-Cyclin E T62+ localization. ( j ) Freshly isolated serum starved synchronized E12.5 NPC were stimulated with ChS for the indicated times and stained for the indicated P-Cyclin E. Percentage of P-Cyclin E + WT NPC plotted versus stimulus duration. ( k ) Interpretation of 3d-3j summarized as a cartoon representing cellular localization of Cyclin E along the inter-nuclear movement of WT VZ-NPC. For further discussion see Supplementary Note 2 . ( l ) Comparison between WT− and ASPM Δ -NPC shown in 3j. ( m ) The NPC described in 3l were also EdU pulse labeled at the indicated times. Percentage of EdU + /P-Cyclin E + cells plotted versus stimulus duration. For high resolution of panels d and i , see Supplementary Fig. 11 . Graphs represent quantified three mice and four sections per mouse. All graphs display mean±s.e.m. * P <0.05, ** P <0.01, *** P <0.0005, **** P <0.00005 by Student’s t -test. Scale bars, 50 μm. Full size image The reduced ASPM Δ Cyclin E detected by western blotting was further established by IHC. In particular, proportions of NPC positive for Cyclin E phosphorylated on residue T62 were significantly reduced ( Fig. 3d,i ) in both G1− and S− phase cells ( Fig. 3e,f ). Proportions of P-Cyclin E T380 were slightly decreased, especially in ASPM Δ G1 cells ( Fig. 3d–f ). Although western blotting depicted reduced level of overall Cyclin E (pan-CycE) ( Fig. 3b ), the largest part of NPC were positive for pan-Cyclin E by IHC ( Fig. 3i ), indicating reduced amount of Cyclin E per cell. This is in line with the significant reduced intensity of staining with anti P-Cyclin E T62 and anti P-Cyclin E T380 Abs, measured in G1− but not in S-phase NPC ( Fig. 3g,h ). Cyclin E in complex with Cdk2 was shown to localize to the nucleus [36] only once beyond the R-point [37] , [38] . Figures 3d,i show that it is the P-Cyclin E T62 that was mainly localizes to the nucleus of G1 cells. S-phase cells, on the other hand, exhibited nuclear Cyclin E of both phosphorylated forms ( Fig. 3d ). Thus, as accumulation of Cyclin E and activity of the Cyclin E/Cdk2 complex reach maximum in late G1 and are essential for passage through the R-point and S-phase entry [39] , the significantly decreased P-Cyclin E T62 in nuclei of ASPM Δ NPC in G1 further signifies postponed passage through the R-point threshold. Detailed analysis of the IHC shown in Fig. 3d–f suggests a sequential phosphorylation of Cyclin E as NPC progress from G1 to S. Starting at mid G1, Cyclin E is mainly phosphorylated on residue T62 before acquiring further phosphorylation on residue T380 at late G1. To support these intriguing observations, in vitro assay was performed on freshly isolated synchronized NPC ( Supplementary Fig. 12a ). At early G1 (3 h), most Cyclin E + WT-NPC were P-Cyclin E T62+ while only 50% were positive for P-Cyclin E T380 ( Fig. 3j,m left panels, Supplementary Fig. 12b ). Past the R-point (13 h), all WT-NPC were P-Cyclin E T62+ . Subsequently, cells became P-Cyclin E T380+ in S-phase (26 h) ( Fig. 3j,k , Supplementary Fig. 12b ). Notably, comparison between WT and ASPM Δ in vitro cultured NPC showed striking resemblance to the in vivo results, that is, a significant decrease in G1− and S− T62 phosphorylation, and a slight decrease in G1− T380 phosphorylation ( Fig. 3l,m ). Furthermore, in vivo and in vitro IHC using pan-CycE Abs exhibited mostly cytoplasmic localization in G1, and dual nuclear and cytoplasmic localization in S ( Fig. 3i , Supplementary Fig. 12b ). Mutant Cyclin E that cannot bind to Cdk2 was shown to localized to the cytoplasm [40] , suggesting that non-phosphorylated Cyclin E in G1 is Cdk2-unbound. Altogether, in vivo and in vitro assessments of Cyclin E levels as NPC proceed from G1 to S, established a crucial ASPM function. Tracking the extent of phosphorylation pinpointed to ASPM regulation of phosphorylated Cyclin E levels, particularly on residue T62, in concert with coordinated passage through the R-point. Aberrant RB-E2F activity along the G1 to S interval In accord with changes in kinase activity ( Fig. 3c ), pRB T821 phosphorylated by the Cyclin E/Cdk2 complex [41] was significantly decreased in ASPM Δ NPC ( Fig. 4a–c ). A related increased levels of pRB S780 , phosphorylated by Cyclin D/Cdk(4/6), were detected ( Fig. 4a ). Particularly significant reduced pRB T821 phosphorylation was observed in ASPM Δ S-phase NPC ( Fig. 4d ). Predicted from the pattern of RB phosphorylation, ASPM Δ NPC displayed significantly reduced endogenous E2F activity ( Fig. 4e ), as well as changes in the relative expression of several E2F target genes ( Supplementary Fig. 13 ). 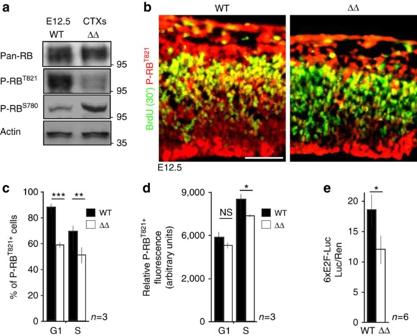Figure 4: ASPM regulates the RB-E2F pathway. (a) Protein lysates of E12.5 telencephalons were analysed for phosphorylated RB. (b) E12.5 embryos were BrdU-pulse labelled for 30 min. Coronal cortical sections were stained for BrdU and the P-RBT821isoform. (c) Chart demonstrating the proportions of P-RBT821+NPC. (d) Chart demonstrating quantification of mean relative fluorescence intensity per cell of P-RBT821staining in G1− and S-phase NPC. Statistically significant decrease in mean fluorescence intensities suggests thatASPMΔS-NPC but not G1-phase cells had become less dense in RB phosphorylated by Cyclin E. (e) 6xE2F-luciferaseplasmid was transfected into isolated E12.5 telencephalic NPC. Luciferase reads, normalized torenillaactivity, represent endogenous E2F activity. Bar graphs represent three mice and four cryosections per mouse that were quantified. All graphs display mean±s.e.m. *P<0.05, **P<0.01, ***P<0.0005 by Student’st-test. Scale bar, 50 μm. Figure 4: ASPM regulates the RB-E2F pathway. ( a ) Protein lysates of E12.5 telencephalons were analysed for phosphorylated RB. ( b ) E12.5 embryos were BrdU-pulse labelled for 30 min. Coronal cortical sections were stained for BrdU and the P-RB T821 isoform. ( c ) Chart demonstrating the proportions of P-RB T821+ NPC. ( d ) Chart demonstrating quantification of mean relative fluorescence intensity per cell of P-RB T821 staining in G1− and S-phase NPC. Statistically significant decrease in mean fluorescence intensities suggests that ASPM Δ S-NPC but not G1-phase cells had become less dense in RB phosphorylated by Cyclin E. ( e ) 6xE2F- luciferase plasmid was transfected into isolated E12.5 telencephalic NPC. Luciferase reads, normalized to renilla activity, represent endogenous E2F activity. Bar graphs represent three mice and four cryosections per mouse that were quantified. All graphs display mean±s.e.m. * P <0.05, ** P <0.01, *** P <0.0005 by Student’s t -test. Scale bar, 50 μm. Full size image Cyclin E- dependent and independent ASPM function To address whether ASPM regulation of CC timing, mitotic cleavage orientation, and fate determination are Cyclin E dependent, E14.5 embryos were transduced in utero with lentivirus harbouring Cyclin E in frame with F2A-mCFP or control mCFP ( Fig. 5a ). Western blot analyses and strong blue fluorescence along the entire cortical wall indicate continuous strong Cyclin E expression ( Fig. 5b,c ). Essentially, ASPM Δ transduced cortices were phenotypically rescued. For the most part, lentiviral-Cyclin E transduction resulted in a complete rescue of late G1 nuclear P-Cyclin E T62 distribution ( Fig. 5c ). Though lentiviral-Cyclin E transduction produced only 10% rescue of whole brain weight ( Fig. 5d ) ( ASPM Δ +mCFP 62.00±0.45 mg; +CycE 68.38±0.88 mg, n =5, P =0.0002 by Student’s t -test), it resulted in a nearly full recovery of the telencephalic vesicle dimensions ( Fig. 5e,f ) ( ASPM Δ +mCFP 4.12±0.028 mm; +CycE 4.35±0.024 mm, n =4, P =0.0005 by Student’s t -test, WT+mCFP 4.37±0.121 mm; +CycE 4.65±0.164 mm, n =6, not significant by Student’s t -test). 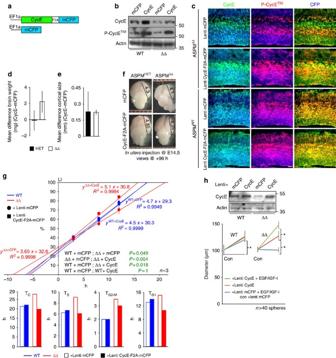Figure 5: Lentiviral-Cyclin E transduction rescuesASPMΔelongated cell-cycle. (a) Schematic diagram of the Cyclin E-F2A-mCFP lentiviral vector. EF1α: elongation factor 1α promoter. F2A: FMDV 2A sequence. Control vector containing only membrane bound Cerulean Fluorescent Protein (mCFP) was employed. (b,c) Expression of pan-Cyclin E and P-Cyclin ET62in E16.5 cortices 48 h afterin uterolentiviral transduction detected by Western blotting and IHC conducted on coronal sections. (d) The effect size between brain weights of E18.5ASPMΔand heterozygous littermates, 96 h followingin uterolentiviral transduction. Guided by Cohen’s modified classification, the difference found forASPMΔembryos is significantd=−0.808. No size effect was found for heterozygous embryos,d=0.028.n=6 (HET+mCFP),n=9 (HET+CycE),n=5 (ASPMΔ+mCFP and +CycE). (e) A direct statistical comparison between the effect sizes of E18.5 cortical lobe length at the anteromedial-posterolateral axis, 96 h followingin uterolentiviral transduction. Guided by Cohen’s modified classification, the difference found for heterozygous embryos is significantd=−0.710, and highly significant forASPMΔembryosd=−3.391.n=5 (HET+mCFP),n=7 (HET+CycE),n=4 (ASPMΔ+mCFP and +CycE). (f) Dorsal views of representative E18.5 brains, lentiviral transduced for 96 h. Dimensions are in millimetres. (g) Cumulative BrdU labeling of E15.5 VZ-NPC that werein uterotransduced with lentiviral vectors 24 h earlier. A 2 × 3 factor ANOVA (groups × survival times) indicates significant main effects between various genotypes and treatments (green). Lower bar graphs depict rescue of theASPMΔelongated TCand its various phases. TCand TSwere deduced directly from the LI graph, TG2+MfromSupplementary Fig. 14c, and TG1=TC—TS—TG2+M. (h) Transduced expression of Cyclin E restored theASPMΔneurospheres lack of response to proliferation stimuli (Fig. 2a). Expression of ectopic Cyclin E in neurospheres 6 days after lentiviral infection was detected by western blotting. All graphs display mean±s.e.m. *P<0.05 by Student’st-test. Scale bar, 50 μm. Figure 5: Lentiviral-Cyclin E transduction rescues ASPM Δ elongated cell-cycle. ( a ) Schematic diagram of the Cyclin E-F2A-mCFP lentiviral vector. EF1α: elongation factor 1α promoter. F2A: FMDV 2A sequence. Control vector containing only membrane bound Cerulean Fluorescent Protein (mCFP) was employed. ( b , c ) Expression of pan-Cyclin E and P-Cyclin E T62 in E16.5 cortices 48 h after in utero lentiviral transduction detected by Western blotting and IHC conducted on coronal sections. ( d ) The effect size between brain weights of E18.5 ASPM Δ and heterozygous littermates, 96 h following in utero lentiviral transduction. Guided by Cohen’s modified classification, the difference found for ASPM Δ embryos is significant d=−0.808 . No size effect was found for heterozygous embryos, d=0.028 . n =6 (HET+mCFP), n =9 (HET+CycE), n =5 ( ASPM Δ +mCFP and +CycE). ( e ) A direct statistical comparison between the effect sizes of E18.5 cortical lobe length at the anteromedial-posterolateral axis, 96 h following in utero lentiviral transduction. Guided by Cohen’s modified classification, the difference found for heterozygous embryos is significant d=−0.710 , and highly significant for ASPM Δ embryos d=−3.391 . n =5 (HET+mCFP), n =7 (HET+CycE), n =4 ( ASPM Δ +mCFP and +CycE). ( f ) Dorsal views of representative E18.5 brains, lentiviral transduced for 96 h. Dimensions are in millimetres. ( g ) Cumulative BrdU labeling of E15.5 VZ-NPC that were in utero transduced with lentiviral vectors 24 h earlier. A 2 × 3 factor ANOVA (groups × survival times) indicates significant main effects between various genotypes and treatments (green). Lower bar graphs depict rescue of the ASPM Δ elongated T C and its various phases. T C and T S were deduced directly from the LI graph, T G2+M from Supplementary Fig. 14c , and T G1 =T C —T S —T G2+M . ( h ) Transduced expression of Cyclin E restored the ASPM Δ neurospheres lack of response to proliferation stimuli ( Fig. 2a ). Expression of ectopic Cyclin E in neurospheres 6 days after lentiviral infection was detected by western blotting. All graphs display mean±s.e.m. * P <0.05 by Student’s t -test. Scale bar, 50 μm. Full size image Restoring adequate levels of Cyclin E into ASPM Δ telencephalic NPC completely corrected their prolonged T C , T S and T G1 ( Fig. 5g ). Similarly, treated ASPM Δ neurospheres responded correctly to growth stimuli ( Fig. 5h ). On the other hand, lentiviral-Cyclin E could not rescue the abnormally oriented ASPM Δ mitoses ( Fig. 6a ). These experiments establish dual mechanisms of ASPM autonomous regulation. Although CC progression is Cyclin E-dependent, mitotic cleavage orientation is Cyclin E-independent. Foremost, lentiviral-Cyclin E transduction was sufficient to confer partial rescue ( ∼ 50%) of the enhanced ASPM Δ CC exit ( Fig. 6b ), suggesting that impaired CC reentry is the combined outcome of both Cyclin E-dependent CC lengthening and Cyclin E-independent abnormal mitotic orientation. Notably, ASPM Δ NPC orientation-independent tendency toward differentiative-neurogenic divisions measured by clonal pair-cell assay ( Fig. 1j ) was completely rescued in infected cells ( Fig. 6c ), further supporting the role of Cyclin E in NPC fate determination. Likewise, ASPM Δ premature exhaustion of the NPC reservoir ( Fig. 1g ) was brought to a standstill by lentiviral-Cyclin E transduction ( Fig. 6d ). 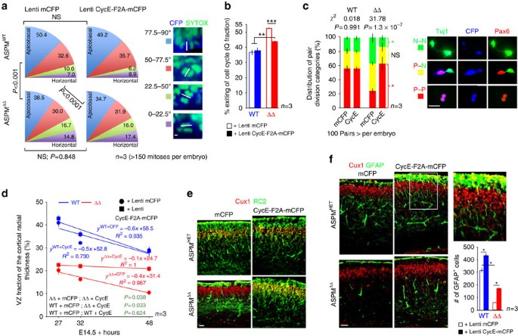Figure 6: Lentiviral-Cyclin E transduction rescuesASPMΔdeficiencies. (a) Distribution of apical mitotic cleavage plane orientation of E16.5 anaphase/telophase cells, lentiviral transduced for 48 h. Χ2statistical analyses confirmed that distribution of horizontal:apicobasal:obliqueASPMΔdivisions was significantly different than control and wasn’t rescue by lentiviral-Cyclin E transduction. Panels on right show representative axes of cleavage plane orientations. (b) Measurement of proportions of C.C exit, 24 h after BrdU pulse labeling and 48 h afterin uterolentiviral transduction. (c) Cyclin E overexpression rescued theASPMΔabnormal P-N cell divisions (Fig. 1j). Freshly isolated E12.5 telencephalic NPC were infected with lentiviral particles. Transgene expression was evaluated 24 h later by CFP, and only blue cells were analysed for clonal pair-fate. (d) Coronal cortical sections, lentiviral transduced at E14.5, were stained for Tuj1. Graph shows best-fit plots of the VZ fractions represented by the Tuj1−region relative to the entire cortical wall radial thickness (seeFig. 1g) versus post transduction survival time. A two-way ANOVA indicates significant main effects between various genotypes and treatments (green). (e) E18.5 coronal cortical sections 96 h following lentiviral transduction stained for Cux1 and RC2. ThoughASPMΔand WT cortices maintain comparable number of RC2+cells,ASPMΔradial glial fibres were not extending throughout the entire cortical plate and terminated at varying positions below the Cux1 layer. (f) E18.5 coronal cortical sections 96 h following lentiviral transduction, stained for Cux1 and GFAP, demonstrating restored astrogenesis. Moreover, lentiviral-Cyclin E transduction into WT cortex accelerated astrogenesis as more radial GFAP+fibers extended into the Cux1 layer (magnification of the boxed area). Bar graph demonstrates GFAP+cell density within a field. All graphs display mean±s.e.m. *P<0.05, **P<0.0005, ***P<0.00001 by Student’st-test. Scale bars, 5 μm (a), 20 μm (c), 50 μm (e,f). Figure 6: Lentiviral-Cyclin E transduction rescues ASPM Δ deficiencies. ( a ) Distribution of apical mitotic cleavage plane orientation of E16.5 anaphase/telophase cells, lentiviral transduced for 48 h. Χ 2 statistical analyses confirmed that distribution of horizontal:apicobasal:oblique ASPM Δ divisions was significantly different than control and wasn’t rescue by lentiviral-Cyclin E transduction. Panels on right show representative axes of cleavage plane orientations. ( b ) Measurement of proportions of C.C exit, 24 h after BrdU pulse labeling and 48 h after in utero lentiviral transduction. ( c ) Cyclin E overexpression rescued the ASPM Δ abnormal P-N cell divisions ( Fig. 1j ). Freshly isolated E12.5 telencephalic NPC were infected with lentiviral particles. Transgene expression was evaluated 24 h later by CFP, and only blue cells were analysed for clonal pair-fate. ( d ) Coronal cortical sections, lentiviral transduced at E14.5, were stained for Tuj1. Graph shows best-fit plots of the VZ fractions represented by the Tuj1 − region relative to the entire cortical wall radial thickness (see Fig. 1g ) versus post transduction survival time. A two-way ANOVA indicates significant main effects between various genotypes and treatments (green). ( e ) E18.5 coronal cortical sections 96 h following lentiviral transduction stained for Cux1 and RC2. Though ASPM Δ and WT cortices maintain comparable number of RC2 + cells, ASPM Δ radial glial fibres were not extending throughout the entire cortical plate and terminated at varying positions below the Cux1 layer. ( f ) E18.5 coronal cortical sections 96 h following lentiviral transduction, stained for Cux1 and GFAP, demonstrating restored astrogenesis. Moreover, lentiviral-Cyclin E transduction into WT cortex accelerated astrogenesis as more radial GFAP + fibers extended into the Cux1 layer (magnification of the boxed area). Bar graph demonstrates GFAP + cell density within a field. All graphs display mean±s.e.m. * P <0.05, ** P <0.0005, *** P <0.00001 by Student’s t -test. Scale bars, 5 μm ( a ), 20 μm ( c ), 50 μm ( e , f ). Full size image The delayed sequence of cortical development within ASPM Δ cortices ( Supplementary Fig. 4a–e ) was restored two days after lentiviral-Cyclin E transduction ( Supplementary Fig. 4f ). By E18.5, as embryonic corticogenesis ceases, even untreated ASPM Δ Cux1 + cells have reached their prospective destination in layers II-IV ( Fig. 6e,f and Supplementary Fig. 4g ). However, these ASPM Δ cortices displayed delayed astrogenesis. ASPM Δ astrocyte progenitors, RC2 + radial glia cells, showed disturbed fiber alignment ( Fig. 6e ). Correspondingly, fewer immature GFAP + astrocytes were observed ( Fig. 6f ). Four days after lentiviral-Cyclin E transduction both deficiencies were restored. The impaired G2/mitosis progression in ASPM Δ cortical germinal layers ( Supplementary Fig. 8 and Supplementary Tables 3 and 4 ), which was further supported by a significantly increased number of PHH3 + cells in mutants ( Supplementary Fig. 14a ), also exhibits Cyclin E dependent and independent modes of ASPM regulation ( Supplementary Fig. 14b–e ). For further discussion into Cyclin A2 expression in ASPM Δ -NPC and the Cyclin A2/ASPM interaction, see Supplementary Fig. 14f–i . ASPM protects Cyclin E from ubiquitination Cyclin E abundance is regulated predominantly at the levels of gene transcription and ubiquitin-dependent proteolysis. The discrepancy between reduced Cyclin E protein levels ( Fig. 3b ) and increased mRNA expression in ASPM Δ NPC ( Supplementary Fig. 13 ) points toward a post-transcriptional ubiquitin-dependent regulation. Accordingly, the high molecular weight smear detected only in ASPM Δ neurospheres treated with the proteasome inhibitor MG132 confirms that ASPM is necessary to protect Cyclin E from ubiquitination ( Fig. 7a ). To determine if administration of proteasome inhibitor could rescue the ASPM Δ abnormalities, settings for in utero introduction of MG132 into developing cortices were calibrated. Administration of MG132 into E15.25 forebrains effectively boosted ASPM Δ Cyclin E levels, especially the ubiquitin-susceptible [42] , [43] , ASPM-regulated P-Cyclin E T62 ( Fig. 7b,c ). Like lentiviral-Cyclin E transduction, MG132 treatment fully reverted the abnormally elongated ASPM Δ T C and T S ( Fig. 7d,e ). In addition, MG132 restored the abnormal excessive ASPM Δ NPC differentiative-neurogenic divisions ( Fig. 7f ), and completely reinstated normal NPC CC exit ( Fig. 7g ). Nevertheless, one must bear in mind that MG132 inhibition of ubiquitin-dependent protein degradation will stabilize many proteins. Thus, the restoration of proper cell cycle is likely to be an additive one through any number of cell cycle regulators. 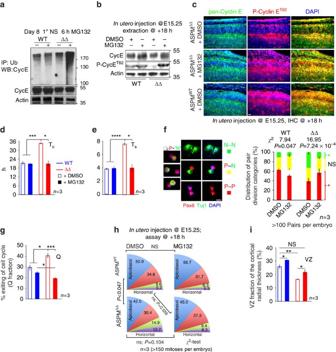Figure 7: ASPM protects Cyclin E from ubiquitination. (a) Primary neurospheres (NS) were treated with the proteasome inhibitor MG132 to preserve ubiquitinated proteins. Lysates, IPed with α-ubiquitin were immunoblotted with α-Cyclin E Abs. (b,c) Western blots and coronal cortical sections of E16 telencephalons, 18 h afterin uteroMG132 administration, analysed with anti pan-Cyclin E and P-Cyclin ET62Abs. (d,e) Charts depicting rescue of theASPMΔelongated TCand TSbyin uteroMG132 administration. Data determined by the double IdU/BrdU labeling procedure. (f) Freshly isolated E12.5 telencephalic NPC analysed for clonal pair-fate, 15 h after MG132 treatment. MG132 caused few P-P pairs to exhibit unusual staining with one Pax6+and another Pax6+Tuj1+. Such pairs were entitled as P-‘N’. (g) Measurement of proportions of E16 NPC exiting the CC 18 h after BrdU pulse labeling coupled within uteroMG132 administration. (h) Histograms depicting cleavage orientation distribution of E16 anaphase/telophase cells, 18 h afterin uteroMG132 administration.Χ2-statistical analysis showed that distribution of horizontal:apicobasal:oblique mitotic divisions of MG132 treatedASPMΔcortices was no longer significantly different than DMSO treated WT controls. (i) E16 Coronal cortical sections, 18 h afterin uteroMG132 administration, were stained for Tuj1. Graph shows the VZ fractions represented by the Tuj1−region relative to the entire cortical wall radial width (seeFig. 1g). All graphs display mean±s.e.m. *P<0.05, **P<0.01, ***P<0.005, ****P<0.001 by Student’st-test. Scale bars represent 20 μm (f), 50 μm (c). Figure 7: ASPM protects Cyclin E from ubiquitination. ( a ) Primary neurospheres (NS) were treated with the proteasome inhibitor MG132 to preserve ubiquitinated proteins. Lysates, IPed with α-ubiquitin were immunoblotted with α-Cyclin E Abs. ( b , c ) Western blots and coronal cortical sections of E16 telencephalons, 18 h after in utero MG132 administration, analysed with anti pan-Cyclin E and P-Cyclin E T62 Abs. ( d , e ) Charts depicting rescue of the ASPM Δ elongated T C and T S by in utero MG132 administration. Data determined by the double IdU/BrdU labeling procedure. ( f ) Freshly isolated E12.5 telencephalic NPC analysed for clonal pair-fate, 15 h after MG132 treatment. MG132 caused few P-P pairs to exhibit unusual staining with one Pax6 + and another Pax6 + Tuj1 + . Such pairs were entitled as P-‘N’. ( g ) Measurement of proportions of E16 NPC exiting the CC 18 h after BrdU pulse labeling coupled with in utero MG132 administration. ( h ) Histograms depicting cleavage orientation distribution of E16 anaphase/telophase cells, 18 h after in utero MG132 administration. Χ 2 -statistical analysis showed that distribution of horizontal:apicobasal:oblique mitotic divisions of MG132 treated ASPM Δ cortices was no longer significantly different than DMSO treated WT controls. ( i ) E16 Coronal cortical sections, 18 h after in utero MG132 administration, were stained for Tuj1. Graph shows the VZ fractions represented by the Tuj1 − region relative to the entire cortical wall radial width (see Fig. 1g ). All graphs display mean±s.e.m. * P <0.05, ** P <0.01, *** P <0.005, **** P <0.001 by Student’s t -test. Scale bars represent 20 μm ( f ), 50 μm ( c ). Full size image The disparity between the partial in utero rescue of Q fraction by lentiviral-Cyclin E ( Fig. 6b ) and the complete rescue by MG132 ( Fig. 7g ) implies that MG132 treatment also affects Cyclin E independent- mitotic orientation dependent- increased ASPM Δ NPC differentiation. Although transduced lentiviral-Cyclin E cortices showed no indication of adjusted ASPM Δ mitotic orientation ( Fig. 6a ), the by far shorter MG132 treatment induced notable, yet statistically insignificant, modification toward normal orientation ( Fig. 7h ). As a result, differences between ASPM WT DMSO-treated and ASPM Δ MG132-treated mitoses became statistically insignificant. In utero MG132 administration most likely affects other converging signalling pathways including the previously shown genetic association between ASPM and β-catenin pathway [44] ( Supplementary Fig. 15 ). Ultimately, ASPM Δ exaggerated depletion of the NPC reservoir ( Fig. 1g ) was stalled by MG132 administration ( Fig. 7i ). ASPM interacts with and stabilizes Cyclin E Cyclin E and ASPM co-localize in several cellular compartments ( Fig. 8a ). Accordingly, ASPM was capable of co-immunoprecipitating the Cyclin E/Cdk2 complex ( Fig. 8b,c ). To examine the part taken by ASPM in Cyclin E turnover, degradation assays were employed. As previously shown [43] , co-expression of Cyclin E with either Fbw7 or Skp2 E3 ubiquitin ligases caused a substantial decrease in the level of Cyclin E protein ( Fig. 8d ). The decrease was partially averted by adding up ASPM ( Fig. 8d ). Correspondingly, overexpression of increasing amounts of ASPM led to a significant decrease of Fbw7− and Skp2-mediated ubiquitination of Cyclin E ( Fig. 8e,f ). Next, the effect of ASPM on Cyclin E association with its ubiquitin E3-ligases was examined. Over-expression of increasing levels of ASPM exceedingly inhibited the association of Cyclin E with Fbw7 and Skp2 ( Fig. 8e,f ). ASPM Δ mice express the truncated 155 kDa ASPM product and an alternatively spliced variant of 205 kDa ( Fig. 9a ). Thus, the variants’ association with Cyclin E was compared with full-length ASPM protein product. All three ASPM isoforms were capable of co-IP with Cyclin E ( Fig. 9a,b ). However, the truncated and the alternatively spliced isoforms were substantially defective in eliminating Cyclin E degradation, as they were not capable of reducing its ubiquitination when expressed at comparable levels ( Fig. 9c ). Thus, full length ASPM is necessary to protect Cyclin E from ubiquitin-mediated degradation. 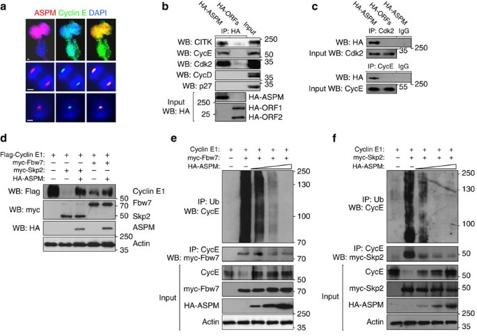Figure 8: ASPM regulation of ubiquitin E3-ligase mediated degradation of Cyclin E. (a) IHC of endogenous Cyclin E and ASPM presents fluctuating levels of diffuse speckled cytoplasmic localization in non-mitotic HEK293T cells. Co-localization was also observed in anaphase spindle poles and the centrosomes as two discrete spots peripheral to the nucleus. Scale bars, 5 μm. (b) HEK293T cells were transfected with HA-tagged human ASPM cDNA. IP was performed on cell extracts with α-HA Abs, and immunoprecipitates were immunoblotted with the indicated Abs. Two HA-tagged unrelated proteins were used to rule out non-specific interactions. ASPM-CITK interaction was employed as a positive control70. Whole cell lysates were used as input. ASPM did not co-IP p27 and Cyclin D. (c) Reciprocal coIP experiments. HA-tagged ASPM transfected HEK293T cell lysates were IPed with α-Cdk2 or α-Cyclin E and immunoblotted with α-HA Abs. Irrelevant HA-tagged cDNAs were used as control, as well as nonspecific rabbit IgGs. (d) Plasmids expressing the indicated tagged cDNAs were co-transfected into HEK293T cells that were not treated with MG132. Lysates were extracted after 48 h and were subjected for Western blotting with the indicated Abs. (e,f) Plasmids expressing the indicated tagged/untagged cDNAs were co-transfected into HEK293T cells. After 36 h cells were treated with MG132 for further 12 h and lysed. Lysates were IPed with α-ubiquitin or α-Cyclin E, and immunoblotted with α-Cyclin E, or α-myc Abs, respectively. 1% of whole cell lysates were used as input. Figure 8: ASPM regulation of ubiquitin E3-ligase mediated degradation of Cyclin E. ( a ) IHC of endogenous Cyclin E and ASPM presents fluctuating levels of diffuse speckled cytoplasmic localization in non-mitotic HEK293T cells. Co-localization was also observed in anaphase spindle poles and the centrosomes as two discrete spots peripheral to the nucleus. Scale bars, 5 μm. ( b ) HEK293T cells were transfected with HA-tagged human ASPM cDNA. IP was performed on cell extracts with α-HA Abs, and immunoprecipitates were immunoblotted with the indicated Abs. Two HA-tagged unrelated proteins were used to rule out non-specific interactions. ASPM-CITK interaction was employed as a positive control [70] . Whole cell lysates were used as input. ASPM did not co-IP p27 and Cyclin D. ( c ) Reciprocal coIP experiments. HA-tagged ASPM transfected HEK293T cell lysates were IPed with α-Cdk2 or α-Cyclin E and immunoblotted with α-HA Abs. Irrelevant HA-tagged cDNAs were used as control, as well as nonspecific rabbit IgGs. ( d ) Plasmids expressing the indicated tagged cDNAs were co-transfected into HEK293T cells that were not treated with MG132. Lysates were extracted after 48 h and were subjected for Western blotting with the indicated Abs. ( e , f ) Plasmids expressing the indicated tagged/untagged cDNAs were co-transfected into HEK293T cells. After 36 h cells were treated with MG132 for further 12 h and lysed. Lysates were IPed with α-ubiquitin or α-Cyclin E, and immunoblotted with α-Cyclin E, or α-myc Abs, respectively. 1% of whole cell lysates were used as input. 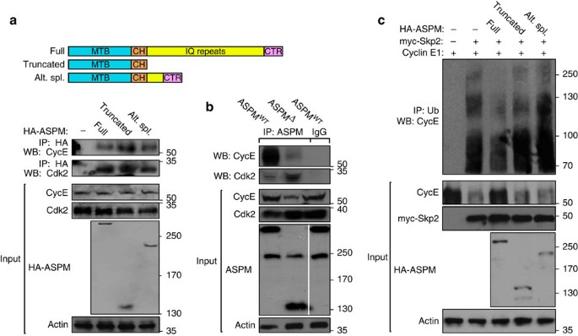Figure 9: ASPM isoforms interaction with Cyclin E and regulation of its ubiquitination. (a) Schematic representation of full length, truncated and alternatively spliced ASPM cDNAs used for the co-IP studies. Plasmids expressing the indicated HA-tagged humanASPMcDNAs were co-transfected with Cyclin E1 into HEK293T cells. After 36 h cells were treated with MG132 for further 12 h and lysed. Lysates were IPed with α-HA and immunoblotted with α-Cyclin E Abs. MTB, microtubule-binding domain; CH, calponin binding domain; IQ, calmodulin binding domain; CTR, C-terminus. (b) co-IP analyses of protein extracts from 5 × E11 WT andASPMΔcortices. Extracts, IPed with α-ASPM Abs, were immunoblotted with Cyclin E and Cdk2 Abs, demonstrating a direct and physiological evidence of endogenous ASPM:Cdk2/Cyclin E association. Data further illustrate the association of endogenous truncated and alternatively spliced ASPM with the Cdk2/Cyclin E complex, as shown inFig. 6a. Note in the input blots, full-length (345 kDa) ASPM proteins were not detected in mutant embryos, whereas the alternate splice variant (205 kDa) expression remained intact. Instead, a truncated (155 kDa) ASPM product was noticed in mutant embryos. (c) Plasmids expressing the indicated HA-tagged humanASPMcDNAs were co-transfected with Cyclin E1 and myc-Skp2 into HEK293T cells. After 36 h cells were treated with MG132 for further 12 h and lysed. Lysates were IPed with α-ubiquitin and immunoblotted with α-Cyclin E Abs. Full size image Figure 9: ASPM isoforms interaction with Cyclin E and regulation of its ubiquitination. ( a ) Schematic representation of full length, truncated and alternatively spliced ASPM cDNAs used for the co-IP studies. Plasmids expressing the indicated HA-tagged human ASPM cDNAs were co-transfected with Cyclin E1 into HEK293T cells. After 36 h cells were treated with MG132 for further 12 h and lysed. Lysates were IPed with α-HA and immunoblotted with α-Cyclin E Abs. MTB, microtubule-binding domain; CH, calponin binding domain; IQ, calmodulin binding domain; CTR, C-terminus. ( b ) co-IP analyses of protein extracts from 5 × E11 WT and ASPM Δ cortices. Extracts, IPed with α-ASPM Abs, were immunoblotted with Cyclin E and Cdk2 Abs, demonstrating a direct and physiological evidence of endogenous ASPM:Cdk2/Cyclin E association. Data further illustrate the association of endogenous truncated and alternatively spliced ASPM with the Cdk2/Cyclin E complex, as shown in Fig. 6a . Note in the input blots, full-length (345 kDa) ASPM proteins were not detected in mutant embryos, whereas the alternate splice variant (205 kDa) expression remained intact. Instead, a truncated (155 kDa) ASPM product was noticed in mutant embryos. ( c ) Plasmids expressing the indicated HA-tagged human ASPM cDNAs were co-transfected with Cyclin E1 and myc-Skp2 into HEK293T cells. After 36 h cells were treated with MG132 for further 12 h and lysed. Lysates were IPed with α-ubiquitin and immunoblotted with α-Cyclin E Abs. Full size image Over the past 2.5 million years our ancestors tripled their brain size with a hallmark expansion of the cerebral cortex, primarily because of an increase in cell number. The majority of cortical neurons originate from proliferating NPC situated in the VZ and SVZ germinal compartments. Essentially, the evolutionary increase in cortical neurons reflects a growing potential of the NPC to undergo more cycles of divisions [45] , [46] . Accordingly, generation of neurons from NPC occurs in a precisely timed fashion. Most of early cortical VZ-NPC undergo symmetric proliferative division to self-renew and expend the progenitor pool. Later on, at mid-corticogenesis, VZ-NPC divide asymmetrically (neurogenic division) to self-renew and to generate either a neuron or an intermediate SVZ precursor. The concluding VZ divisions as well as SVZ-NPC undergo symmetric neurogenic division to generate two neurons [3] , [16] , [18] . However, comprehensive understanding of the mechanisms that regulate the switch from symmetric proliferative to asymmetric neurogenic to symmetric neurogenic cell division is lacking. Data illustrated here confirm the link between CC duration and spatio-temporal control of the number of emerging neurons. While in faster cycling NPC, division mode appears to correlate with cleavage plane orientation independent of CC duration, the frequency of differentiative divisions increases only among NPC whose CC exceeds a threshold, in accordance with the G1- phase length hypothesis [15] , [16] . The present study provides surprising new insights to the process by which phase length affects NPC fate decisions. Though ASPM Δ NPC exhibit elongated CC, the lengthening could not be solely attributed to a G1 increase, as progression through S− and G2/M-phases were also delayed. Especially surprising was the finding that significant lengthening of the G1 occurred only in late (E16.5) ASPM Δ NPC. Although G1 duration of early ASPM Δ NPC was normal, comprehensive measurements established that the transition through the G1− R-point was significantly postponed. The lack of reliable markers presented a challenge to distinguish between early and late G1-phases. However, the transfer of phosphorylated Cyclin E isoforms into the nucleus proved to be reliable indicative tool. This novel method corroborated the finding of delayed passage from the intrinsic and extrinsic signals-dependent early G1 to mitogen-independent late G1. Hence, in compliance with ASPM peaking during G1 (ref. 47 ), ASPM Δ G1-NPC linger uncommitted throughout a longer episode of susceptibility to mitogenic differentiation signals ( Fig. 10 ). 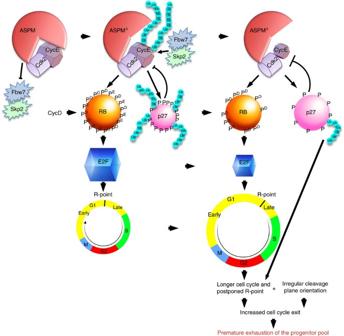Figure 10: Diagram illustrating the proposed model for ASPM regulation of the Skp2/Fbw7− Cyclin E/Cdk2− RB− E2F− R-point pathway with consequences for regulation of asymmetric stem cell division in parallel to formerly reported control of mitotic spindle orientation. . Figure 10: Diagram illustrating the proposed model for ASPM regulation of the Skp2/Fbw7− Cyclin E/Cdk2− RB− E2F− R-point pathway with consequences for regulation of asymmetric stem cell division in parallel to formerly reported control of mitotic spindle orientation. . Full size image Proper CC progression depends on strict management of Cyclin E/Cdk2 levels and activities. Correspondingly, Cyclin E abundance oscillates during normal CC attaining a maximum level of expression in late G1 (ref. 39 ). However, studies have demonstrated that Cyclin E also controls mitotic progression (see references in Supplementary Fig. 14 ), and S-phase progression and completion in a pRB/E2F independent manner [48] , [49] . Accordingly, it has been demonstrated that the expansion of the NPC reservoir correlates with the time spent by the cells during S-pahse [17] . In addition to gene transcription, Cyclin E abundance is controlled at the level of ubiquitin-dependent proteolysis. Various modes of regulations direct Cyclin E degradation including ubiquitination by at least two E3-ligases (Fbw7 and Skp2) associated with phosphorylation on at least four different sites, T62, S372, T380 and S384, by at least two kinases (Gsk3 and Cdk2) [36] , [37] , [40] , [42] , [43] , [50] , [51] , [52] . Cyclin E contains two Cdc4-phosphodegron motifs that direct Fbw7 binding and stimulate Cyclin E ubiquitination and degradation [53] . The T380-containing degron is regarded as the dominant Cyclin E degradation signal making more extensive high-affinity contacts with Fbw7, whereas the T62 site is a weaker sub-optimal degron [40] , [42] , [43] , [50] , [54] , [55] . Therefore, the T380-containing degron has been considered more physiologically significant. Thus, the difference of P-CycE T380 signal intensity between WT and ASPM Δ NPC is expected to be bigger than P-CycE T62 . However, previous studies have shown that ablation of the T380 degron did not fully stabilize Cyclin E [56] . Also, mutation of T62 reduced the extent of T380 phosphorylation [43] , suggesting an indirect effect of the T62 degron on Cyclin E degradation through the T380 degron. Otherwise, the two-phosphodegron motifs might function as independent redundant pathway- or tissue-specific constituents of Cyclin E degradation. A previously unknown pattern of sequential Cyclin E phosphorylation, as NPC progress along G1− into S-phase, is demonstrated here ( Fig. 3j–m ). Initially, at mid G1, residue T62 is predominantly phosphorylated followed by added phosphorylation on T380. Accordingly, we propose that in addition to independent spatial function, the two-phosphodegron motifs might also exhibit independent temporal function. As NPC progress along the G1-phase, Cyclin E is first phosphorylated at T62 subjecting it to ubiquitination and degradation. By the time T380 is being phosphorylated, most of Cyclin E has already been degraded. Hence, a comparison between P-CycE T380 and P-CycE T62 signal intensities in WT− and ASPM Δ -NPC showed similar decrease ( Fig. 3g ). Cyclin E phosphorylation on T380 does not require Cdk2 (ref. 40 ), suggesting that Cdk2 affects Cyclin E turnover primarily via T62. Thus, T62 being the earliest phosphorylated residue with a sustained prominence throughout the G1 to S interval is reminiscent of Cdk2 being Cyclin E immediate partner. Clear partitioning of ASPM functions into two autonomous mechanisms was achieved by in utero lentiviral-Cyclin E transduction experiments. Cyclin E-dependency was established by an absolute reinstatement of the aberrant mutant CC. In contrast, mitotic cleavage regulation proved to be Cyclin E-independent due to ineffective rescue of orientation irregularity. On the whole, Cyclin E partial rescue of the ASPM Δ increased rate of differentiation corroborates that ASPM regulation of NPC fate is a combination of both Cyclin E-dependent CC duration, and Cyclin E-independent cleavage plane orientation ( Fig. 10 ). Interestingly, lentiviral-Cyclin E transduction into heterozygous telencephalons resulted in an insignificantly increased cortical lobe length at the anteromedial-posterolateral axis ( Fig. 5e,f ) in correlation with no apparent acceleration of the CC and its various phases ( Fig. 5g ). Moreover, lentiviral-Cyclin E transduced WT neurospheres were not hypersensitive to proliferation stimuli ( Fig. 5h ). Consequently, the NPC reservoir of lentiviral-Cyclin E transduced WT cortices declined in the same pace as control ( Fig. 6d ). On the other hand, lentiviral-Cyclin E transduced ASPM Δ NPC displayed significantly shorten CC, primarily due to shorter T G1 , even in comparison to WT. Furthermore, stimulated lentiviral-Cyclin E transduced ASPM Δ neurospheres grew faster then WT. The Cyclin D-Cyclin E-Rb-E2F pathway functions as a bistable switch regulating the R-point upon the cell commitment to proliferation independently of external stimulation. The nature of a bistable switch mechanism is based on high-threshold, low-maintenance characteristics. First, high threshold of stimulation is established to guarantee preconditions for fully implemented proliferation followed by a low-maintenance requirements to ensure that the cycle is completed once initiated, even in the absence of continuous stimulation. Once turned ON by adequate stimulation, E2F memorize and sustain this ON state independently of constant stimulation [57] . At the beginning of G1, E2F is bound to and repressed by RB. With sufficient stimulation, activity of Cyclin D/Cdk4,6 is induced to launch RB phosphorylation and to relieve its repression of E2F. E2F activates the transcription of Cyclin E, which complexes with Cdk2 to further phosphorylate and completely remove RB repression, establishing a positive-feedback loop, which is a hallmark of a bistable switch. Hence, the stably balanced WT R-point is not affected by addition of Cyclin E due to several positive feedback circuits (also including the mutual inhibition between Cyclin E/Cdk2 and p27 Kip1 loop). ASPM Δ R-point, on the other hand, is unstable and therefore responds more erratically to external stimulations such as the lentiviral-Cyclin E transduction. The absence of change in the mode of division after lentiviral-Cyclin E transduction into WT-NPC ( Fig. 6b,c ) stands at odds with previously published results [22] . A number of procedural variations between the two assays might result in the discrepancy. Namely, the electroporation method used by Pilaz et al. selectively targets S−, G2−, and M-phase VZ-NPC with a very low efficiency in G1 cells. This is not the case with lentiviral infection that targets all cells, irrespectively of their cycling status. Nonetheless, while Pilaz et al. demonstrated that cumulative S phase labelling was inappropriately used for measuring CC kinetics in synchronous electroporated population [21] , lentiviral mediated gene transfer yielded >99% overexpression efficiency ( Fig. 5c ), and therefore is compatible with any S-phase labelling technique. Since all the defined microcephaly proteins reside at centrosomes or spindle poles, the predominant model for the etiology of microcephaly has emphasized on spindle organization, stability, and orientation as well as centrosome function, assembly, stability, maturation and amplification [58] , [59] . Therefore, the most studied basis for microcephaly involves disrupted spindle orientation and altered symmetric division of NPC, leading to depletion of the progenitor pool and increased neuronal differentiation [28] , [59] , [60] . However, current studies have identified more diverse cellular grounds for microcephaly including, DNA damage response and repair [60] , [61] , [62] , [63] , transcriptional regulation [61] , [63] , [64] , centriole biogenesis [65] , mitotic arrest [58] , [59] , [66] , cell death [59] , [65] , [66] , [67] , ciliogenes [58] and lipid transport [68] . Our study adds the ubiquitin-Cyclin E-Rb-E2F as an additional cellular pathway that plays a major role in the etiology of microcephaly. Mouse breeding Mice were maintained in pathogen-free conditions. All surgical intervention and subsequent care and treatment were in strict accordance with the PHS Policy on Humane Care and Use of Laboratory Animals and the University of Utah IACUC guidelines. Tissue processing Brains of E16.5-E17.5, P4 and 8–10-weeks-old mice were removed from the skull and fixed by immersion in 4% paraformaldehyde (PFA) for 3.5 h at 4 °C. Younger then E16.5 embryos were decapitated and the entire heads were fixed. Samples were washed three times in PBS before cryoprotected in 10%, 20 and 30% (v/v) sucrose gradient in PBS at 4 °C and embedded in OCT tissue-freezing medium (Tissue-Tek). Tails (postnatal) or trunk (embryo) samples were collected for genotyping. Immunofluorescence Sections were permeabilized and blocked in PBST (1 × PBS, 0.5% (v/v) Triton X-100) containing 10% NGS for 1 h at 4 °C. Primary Abs were incubated overnight at 4 °C in PBST with 5% NGS and secondary Abs were incubated in the same buffer for 1–2 h at room temperature (RT). Nuclei were stained with DAPI. Terminal deoxynucleotidyl transferase dUTP nick end labelling (TUNEL) was performed using the in situ cell death detection kit (Roche BioSciences). Slides were mounted in Flouromount-G anti-fade reagent (SouthernBiotech). For pulse-chase experiments 5-Bromo-2’-deoxyuridine (BrdU dissolved in 0.007 N NaOH, 0.9% NaCl), 5-Iodo-2′-deoxyuridine (IdU dissolved in 0.014 N NaOH, 0.9% NaCl) and 5-Chloro-2’-deoxyuridine (ChdU dissolved in PBS) (Sigma-Aldrich) were injected intraperitoneally (50 μg g -1 ) and chased for times specified. Sections were air dry for 1 h at RT, followed by 20 min incubation in acetone at 4 °C and air dry again for 1 h at RT. Next, the sections were washed in PBST and antigen was unmasked by boiling for 13 min in 10 mM Citrate buffer (pH 6). Once solution had cooled down to RT, sections were washed in PBST and treated for 45 min with 2 N HCl/0.1% Triton X-100 in PBS at 37 °C. After extensive washes, the sections were blocked and incubated with the respected Abs as before. In case of double staining with one Abs being an S-phase tracer (IdU/BrdU/ChdU), after cooling down from boiling in Citrate buffer, sections were blocked and incubated overnight with the non-tracer Abs at 4 °C. Following incubation with the appropriate secondary Abs and adequate washing, sections were postfix with 8% PFA in PBS for 20 min at 4 °C before proceeding to the HCl treatment as described above. For NPC and HEK293T immunostaining, cells were fixed in ice-cold 4% PFA solution for 30 min followed by ice-cold methanol for 5 min before successively treated with primary and secondary Abs. For Abs and dilutions, see Supplementary Table 6 . Determination of basal mitoses cleavage plane orientation SYTOX (Molecular Probes)-stained chromosomes in metaphase and anaphase/telophase were sorted according to the angle of the cleavage plane relative to the ventricle surface (VS). Cleavage plane was defined as horizontal (0–30°), that is, the mitotic spindle aligned perpendicular to the VS, oblique (30–60°), or vertical (60–90°), that is, mitotic spindle aligned parallel to the apical-basal axis of the VS. To simultaneously identify chromosomes and the entire framework of the basal mitoses sections were co-stained for Alexa Flour 546 phalloidin (Invitrogen). In vitro culture of neural progenitors NPC isolation . E12.5 telencephalic lobes were dissected and digested for 30 min at RT with 500 U ml -1 papain (Worthington) and 100 U ml -1 DNase I (Fermentas) in dissociation medium (DMEM/F12 supplemented with sodium pyruvate, non-essential amino-acids, L -glutamine (GibcoBRL) and 5 mM N -acetyl-cysteine (Sigma-Aldrich)) with rocking. Enzymatic digestion was stop by addition of DMEM/F12 medium. Tissue was disintegrated into a single cell suspension by gentle pipetting. Cells were passed though a 45 μm nylon screen. Neurospheres Cells were seeded at clonal density (5,000 cells cm -2 1.3 cells μl -1 ) onto ultra low attachment multiwell plates (costar) in Neurosphere medium (DMEM/F12 supplemented with sodium pyruvate, L -glutamine, penicillin/streptomycin, N2, B-27, 1 mM N -acetyl-cysteine, 15% chick embryo extract (Invitrogen) and 20 ng ml -1 human basic fibroblast growth factor (bFGF; R&D Systems) was added daily). Neurospheres were incubated in the presence of 20 ng ml -1 epidermal growth factor (EGF) and 20 ng ml -1 insulin-like growth factor (IGF-I) (R&D Systems) to stimulate proliferation. Diameters of single neurospheres were measured after 7 days of culture. Seven day-old primary neurospheres were triturated to yield single cell suspensions then grown for 7 additional days to assess sizes of secondary neurospheres. Images were acquired using Leica EL6000 microscope and captured with Digital Photo Professional version 3.3.1 software (Canon Inc.). Pair-cell analysis Single cells were plated at clonal density (30–40 cells well -1 ) into poly- L -lysine-coated 16-well glass slide (Nunc) in serum-free medium (DMEM with L -glutamine, sodium pyruvate, B-27, N2, 1 mM N -acetyl-cysteine and 10 ng ml -1 bFGF). Pair-cells were identified at 24 h, washed, fixed and stained for Pax6 and Tuj1. For secondary pair-cell analysis, freshly isolated single cells were plated into 60 mm poly- L -lysine-coated plates in Neurospheres medium for 24 or 48 h, before applying enzymatic detachment (papain), three washes and re-plating for additional 24 or 48 h as describe. P-P pairs were assessed as being Pax6 + /Pax6 + and TuJ1 − /TuJ1 − . N-N pairs were assessed as being Pax6 − /Pax6 − and TuJ1 + /TuJ1 + . P-N pairs were assessed as being Pax6 + /TuJ1 − and Pax6 − /TuJ1 + . For Abs and dilutions, see Supplementary Table 6 . In utero lentiviral transduction An E14.5 pregnant dams were anesthetized with 2.5% Avertin (1.8 cm 3 g -1 , ip injection). The anesthetized mice were placed on a 37 °C heating pad (FHC, Bowdoin, ME) and the depth of anesthesia was evaluated by examination of pinch withdrawal, eyelid reflex, vibrissae movements and respiration rate. Abdominal hair was removed and skin surface was disinfected with 10% povidone-iodine (Vetone) and sterilized with 70% ethanol. Embryos were taken out of the peritoneal cavity through a 1 cm midline incision and attentively kept moist while out of the peritoneum. 1 μl of lentiviral solution, diluted 1:100 in 0.05% Fast Green (SIGMA) in HBSS, was administered into the embryonic lateral ventricles through the uterine wall using a Hamilton syringe (#95) and a 34 gauge beveled needle (NF34BV, WPI) adjusted with a modified gasket adaptor (NF GSK-5, WPI). The uterus was placed back into the peritoneal cavity and lavaged with sterile PBS. Abdominal musculature and skin were closed using Reflex 9 stainless steel wound clips. Dams were placed on their back in the cage at 37 °C and wounds were administrated with 0.5% Marcaine. In utero proteasome inhibitor administration E15.25 pregnant dams were anesthetized and treated as before. MG132 (50 mM, stock) was diluted to 5 μM with 0.05% Fast Green in HBSS. Similarly, DMSO was diluted 1:10,000 with 0.05% Fast Green in HBSS. Embryos lateral ventricles were injected with 0.4 μl solution. All procedures were terminated within 18 h. These carefully calibrated setting enabled analysis without apparent increased cell death. Transcription activity of endogenous E2F Freshly isolated E12.5 telecephalic cells maintained in neurosphere medium were allowed to attach to poly- L -lysine coated plates for 8 h before transfected using lipofectamine (invitrogen) according to manufacturer’s directions. The Luciferase and Renilla assays were performed 36 h after transfection (Promega) according to manufacturer’s directions and measured on a luminometer. The E2F transcription reporter, 6xE2F-luciferase , construct contains the following sequence 5′-TTTCGCGCTTAA′TTTCGCGCCAAA′CG CGTGCTAGC′TTTCGCGCCAAA′TTTCGCGCTTAA′TTTCGCGGCAAA′TATATAAT-3′ inserted into pGL3 vector (Promega) in front of the luciferase coding sequence. It includes the following six E2F binding sites in tandem: 12mer from position −68 of the E2AE1 gene in the adenovirus 2 genome, position −10 of the mouse DHFR gene, second E2AE1 bonding site, second DHFR binding site, third E2AE1, and position −46 of the mouse E2F1 gene before TATA box. CMV-Renilla construct was used for normalizing the efficiency of the transfection. Kinase assays E12.5 telencephalic lobe extracts were incubated ON at 4 °C with saturating concentrations of Cyclin E, Cdk2, or Cyclin D1 Abs. Immune complexes were collected by incubation with Dynabeads Protein G (invitrogen) for 1 h at 4 °C, and equilibrated on kinase buffer (50 mM TrisHCl pH7.5, 20 mM EGTA, 10 mM MgCl 2 , 1 mM DTT, 1 mM β-glycerolphosphate). For the kinase assays, 10 μl of kinase reaction mixture (0.4 mM ATP pH 7.5, and 10 mCi [γ- 32 P]ATP (Amersham Pharmacia)) in kinase buffer containing substrate (2.5 μg of histone-H1 (Sigma-Aldrich) for Cyclin E and Cdk2, and 0.2 μg of soluble GST-pRb fusion protein (Santa Cruz Biotechnology) for Cyclin D1, was added to the immunoprecipitated complexes. After 30 min of incubation at 37 °C, reactions were stopped by adding 5 μl of Laemmli loading SDS buffer and heating at 100 °C for 10 min. Labelled proteins were resolved by 15% SDS–PAGE. Gels were incubated twice in 20% methanol; 10% glycerol solution before dried on 3 mm paper at 50 °C with vacuum. Images were acquired on Typhoon TRIO+ imaging system (Amersham). For Abs and dilutions, see Supplementary Table 6 . Semi quantitative RT-PCR analysis Isolated total RNA (Tri-Reagent MRC) was reverse transcribed using First Strand cDNA Synthesis kit (Fermentas). For primer sequences, see Supplementary Table 5 . Plasmids To generate HA-hASPM expression plasmid, the human ASPM coding region was amplified by PCR from total human fetal brain cDNA (BioChain Institute, Inc.) and cloned into HA containing plasmid under CAG promoter. To generate hCyclin E1, myc-hSKP2 and myc-hFBW7 expression plasmids the human respective coding regions were amplified by RT-PCR from HEK293T total RNA extracts and cloned into non-tagged or myc containing plasmids, respectively under CAG promoters. The pcDNA3-myc-wt-mCycE, pcDNA3-myc-mCycE T62G , pcDNA3-myc-mCycE T380G plasmids were obtained from Genscript. Coimmunoprecipitation Lysates of MG132 treated neurospheres (20 μM, Sigma-Aldrich) or HEK293T cells transiently expressing HA-tagged respective proteins were incubated overnight at 4 °C with anti-HA or anti-Ub Abs, respectively, cross-linked (dimethyl pimelimidate) beforehand to Dynabeads Protein G (invitrogen). Adequately washed bound material was subsequently eluted by 50 mM Glycine (pH 2.8) and boiled for 10 min. Standard western blotting procedure was used to analyse the immunoprecipitants and input samples. For Abs and dilutions, see Supplementary Table 6 . Uncropped images of blots are shown in Supplementary Figs 16 and 17 . Post-blot images are shown in Supplementary Fig. 18 . Statistical analysis and microscopy All cell counting, tilt classification, dimension and immunofluorescence intensity measures were made without the experimenter being aware of the subject genotype. Images were acquired using Zeiss Axiovert 200 M microscope and captured with Slidebook software (Intelligent Imaging Innovations). Analyses were performed on randomly collected 4–10 non-consecutive serial coronal sections taken from approximately the mid-hemisphere level corresponding to the primordial primary somatosensory cortex. Counts were performed manually in a fixed area of 500 μm in its medial-lateral dimension and 6 μm (corresponding to section thickness) in its rostral-caudal dimension for all the different applications. Results were averaged per animal. No statistical method was used to predetermine sample size since there were no attrition or exclusion of samples. To distinguish between independent data points, experiments were biologically repeated three to four times from animals of at least two different litters. Acquired data was normally distributed and variation within each experimental group was similar. Statistical tests were used to compare data and their P values are indicated in the figure legends. Data were analysed with Excel software using Student’s t -test (Microsoft). P values (2-tailed) <0.05 were considered statistically significant. For multiple group analyses, a two-way ANOVA (JMP 8 software) or Χ 2 -square (Excel software) were applied. How to cite this article: Capecchi, M. R. & Pozner, A. ASPM regulates symmetric stem cell division by tuning Cyclin E ubiquitination. Nat. Commun. 6:8763 doi: 10.1038/ncomms9763 (2015).